Dissecting a heterotic gene through GradedPool-Seq mapping informs a rice-improvement strategy Hybrid rice breeding for exploiting hybrid vigor, heterosis, has greatly increased grain yield. However, the heterosis-related genes associated with rice grain production remain largely unknown, partly because comprehensive mapping of heterosis-related traits is still labor-intensive and time-consuming. Here, we present a quantitative trait locus (QTL) mapping method, GradedPool-Seq, for rapidly mapping QTLs by whole-genome sequencing of graded-pool samples from F 2 progeny via bulked-segregant analysis. We implement this method and map-based cloning to dissect the heterotic QTL GW3p6 from the female line. We then generate the near isogenic line NIL-FH676:: GW3p6 by introgressing the GW3p6 allele from the female line Guangzhan63-4S into the male inbred line Fuhui676. The NIL-FH676:: GW3p6 exhibits grain yield highly increased compared to Fuhui676. This study demonstrates that it may be possible to achieve a high level of grain production in inbred rice lines without the need to construct hybrids. Rice heterosis, or hybrid vigor, refers to the increased yield in a hybrid offspring compared to its inbred parental lines. The rice hybrid varieties typically display a grain yield advantage of 10–30% over their parents [1] . Beginning with the first commercial hybrid maize varieties in the 1930s [2] , and the development of hybrid rice in the early 1970s in China [3] , exploitation of heterosis in crop plants has achieved remarkable yield advantages over traditional breeding of inbred lines. To date, hybrid breeding that combines superior alleles from both parental lines to generate a better F 1 variety is still one of the fastest and most efficient approaches in the breeding of rice as well as in many other crops. However, modern hybrid breeding relying on random crosses between diverse varieties and comprehensive phenotypic selection is still labor-intensive and time-consuming. In the efforts to uncover the genetic basis of heterosis [4] , [5] , there are several non-mutually exclusive hypotheses for heterosis, i.e., dominance, overdominance and epistasis [6] , [7] , with evidences from many molecular genetic experiments that have been performed [8] , [9] , [10] , [11] , [12] , [13] , [14] . In recent work, the genetic basis of heterosis with regard to rice grain yield has been explored by an integrated genomic approach to construct a genome map of 1495 elite hybrid rice varieties and the in-depth genetic analyses on 17 F 2 populations [15] , [16] . The results showed that a small number of genomic loci from female parents explained a large proportion of the yield advantage of hybrids over their male parents of elite inbred varieties. For most of the heterosis-related loci identified, dominance or incomplete dominance of heterozygous loci plays an important role. Therefore, by optimizing cross design, characterization and dissection of heterotic genes and their allelic distribution in diverse germplasms will greatly enhance genetic improvement of rice. Several important high-yielding or heterosis-related genes have been characterized, such as the Ghd7 gene [17] from the male parent (restore line) MH63 and the Ghd8 gene [18] , [19] from the male lines HR5 and 9311. In contrast, yield-associated heterotic genes from female parents (male-sterile lines) remain largely unknown in rice. Genetic mapping for complex agronomic traits through linkage analysis or genome-wide association study (GWAS) showed its great power in the last few decades [20] , [21] , [22] , [23] , [24] , [25] , which will help to identify the heterotic genes from female parents in hybrid rice. In this study, to accelerate the genetic mapping processes, we develop a quantitative trait locus (QTL) mapping approach, GradedPool-Seq (GPS), that combines high-throughput sequencing with bulked-segregant analysis (BSA). This method is to score and assign F 2 generations derived from a distant cross of parental lines exhibiting contrasting phenotypes into three or more graded groups based on their measured phenotypic values. Compared to previous methods using BSA coupled with whole-genome sequencing, such as MutMap [26] , SHOREmap [27] , next-generation mapping [28] and QTL-seq [29] , [30] , the GPS approach has the advantage of performing genetic mapping to simultaneously detect several QTLs at high resolution (~400-kb) by only requiring F 2 population. Furthermore, we can assess multiple phenotypic traits using one F 2 population. This method also allows us to rapidly identify heterotic genes. Benefitting from the robust GPS method coupled with follow-up experiments, we identified and validated a heterotic gene, GW3p6 (OsMADS1) , from the female line (male-sterile line), that contributed greatly to 1000-grain weight and grain yield per plant in an elite hybrid rice variety Guang-Liang-You-676 (GLY-676). Notably, the near-isogenic line (NIL) NIL-FH676:: GW3p6 produced by introgressing the GW3p6 allele from the female line (Guangzhan63-4S, hereafter as GZ) into the male line (Fuhui676, hereafter as FH) exhibit grain yield highly increased compared to FH plants. Rice hybrid breeding is currently hindered by bottlenecks of inefficiency and directionlessness [31] , and the results of this study inform that it can open the door to achieving a high level of grain production using inbred lines instead of generating hybrids. Development of the GPS method To rapidly identify QTLs for complex traits, we developed a method to map QTLs by directly sequencing graded-pool samples (GPS) from F 2 progeny using modified BSA. The GPS procedure, including data obtainment, the filtering process, and statistical analysis, can be explained using plant height phenotype as an example (Fig. 1 , Supplementary Fig. 1 ). To begin with, the mapping populations were developed from a cross between two genetically distant parental lines, one with a higher and the other with a lower phenotypic value of plant height, followed by subsequent self-pollination. Given that the parental lines display contrasting target phenotypes controlled by multiple genes, we predicted that the phenotypic variations in plant height among the F 2 progeny will follow a pattern close to the normal distribution. By assessing plant height in each individual, we classified the F 2 population into several graded bulks (three graded bulks in the graphic example) from the highest to lowest bulk according to their frequency distribution, as opposed to the two phenotypic tails used in BSA (Fig. 1a ). We selected 100 to 150 individuals from each bulk in equal mixed DNA samples with sufficient genomic coverage (average 0.5×–1× per individual) for sequencing to guarantee sequencing accuracy; selection of 20–30% of the total individuals as a bulk is recommended. Next, the sequence reads of each bulk were aligned against the reference genome sequence to estimate allelic frequencies. We assumed that the depth at each single nucleotide polymorphism (SNP) was 100×. If a variance is not related to the phenotype, it would present 50% reference reads and 50% alternate reads in all three bulks; related SNPs would show great distinction in reference reads to alternate reads between the Grade 1 and Grade 3 bulks (Fig. 1b ). Fig. 1 The procedure of the GPS method. a F 2 populations were generated by crossing two parent lines with distinct background and showed vastly different in plant height, followed by the self-pollination of F 1 generation. Through the observation of plant height, F 2 populations were classified from the highest to lowest bulk according to their frequency distribution. The letters M and F indicated the male parents and female parents, respectively. b The sequence reads of each bulk were aligned against the reference genome sequence to estimate allelic frequencies. We assumed that the depth at each SNP was 100×. If a variance was not related to the phenotype, it would present 50% reference reads and 50% alternate reads in all three bulks (right), whereas the related SNP would have great distinction of the ratio of reference reads to alternate reads among three bulks (left and middle). c Data analysis included Ridit analysis and reducing background noise approach. Several associated genetic intervals were mapped and indicated as red four-pointed star Full size image Data analysis was carried out as presented in Fig. 1c . We performed the statistical test, Ridit analysis, which adequately examines and analyses ordinal data [32] , for each variant to compute its p value. Theoretically, if a variant is closely linked to a phenotype-related gene, its p value will be relatively small; however, it is not enough to predict the causative variant due to a large quantity of background noise in SNP calling by the distantly genetic cross. Consequently, background noise reduction must be taken into consideration. The noise-reduction algorithm we implemented in this study was a non-overlap sliding window approach, calculating the ratio of the number of statistically significant variants beyond the set threshold to the total number of variants in a defined genomic interval (~400 kb). Thus, we sought the interval with the largest ratio, i.e., SNPs clusters with significant p values in the highest proportion. The relationship between the ratio and chromosomal intervals reveals those genomic regions where QTLs associated with plant height are most likely to be located. To assess its efficiency and robustness, we applied the GPS pipeline to identify QTLs underlying four agricultural traits (heading date, plant height, flag leaf angle and tiller angle). Multiple QTLs related to these four traits were mapped by GPS, and we focused on the phenotype of plant height. Three F 2 populations of ~400 rice individuals were generated by crossing parental lines exhibiting a distinct plant height phenotype. 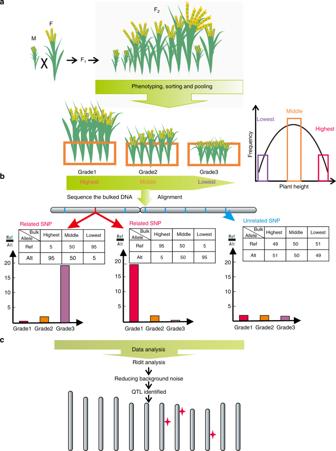Fig. 1 The procedure of the GPS method.aF2populations were generated by crossing two parent lines with distinct background and showed vastly different in plant height, followed by the self-pollination of F1generation. Through the observation of plant height, F2populations were classified from the highest to lowest bulk according to their frequency distribution. The letters M and F indicated the male parents and female parents, respectively.bThe sequence reads of each bulk were aligned against the reference genome sequence to estimate allelic frequencies. We assumed that the depth at each SNP was 100×. If a variance was not related to the phenotype, it would present 50% reference reads and 50% alternate reads in all three bulks (right), whereas the related SNP would have great distinction of the ratio of reference reads to alternate reads among three bulks (left and middle).cData analysis included Ridit analysis and reducing background noise approach. Several associated genetic intervals were mapped and indicated as red four-pointed star According to the phenotypic value, we categorized the F 2 lines into several ordinal classes from highest to lowest (Supplementary Table 1 ), followed with sequencing of the pools. After aligning the sequence reads to the reference sequence (IRGSP build 4) via BWA software [33] and variant calling using GATK [34] , we obtained genome-wide SNP information to conduct filtering procedure step by step, which filtered out at least half of the variants or SNPs with low-quality and inappropriate depth. Next, we calculated p value using Ridit analysis at each variant’s position and generated a p value plot corresponding to its genomic position (Supplementary Fig. 2a, c, e ). Nevertheless, determining a small and precise region was complicated by enormous background noise. Thus, reducing background noise is indispensable. After implementing a noise-reduction algorithm, we narrowed down the interval to 400 kb and successfully localized several intervals harboring causative genes from the ratio plot (Supplementary Fig. 2b, d, f ). Among the identified intervals, Ghd7 and sd1 (refs. [17] , [35] ) are exactly located in our mapping regions, and the GW6a gene [36] is located in a position closely adjacent to the mapping interval on chromosome 6. These results demonstrate that the GPS method can rapidly and accurately identify QTLs underlying the target traits. Other identified genetic regions not consistent with any known genes might harbor new QTLs, although further verification is needed. Moreover, we evaluated the power of GPS to detect regions responsible for heading date, tiller angle and flag leaf angle. The phenotype categories for the F 2 generations are listed in Supplementary Table 1 , and ratio plots are presented in Supplementary Fig. 3 . The results for these four agronomic traits all suggested robust applications of our method (Table 1 ). We then performed GPS to analyze Takagi et al.’s data [29] , comparing with another WGS-BSA method. The results showed consistency with their results, and our mapping region of causal genes was narrowed to 0.4 Mb (Supplementary Fig. 4 ). Additionally, we explored the whole procedure of our approach in depth, especially the influence on results when changing experimental variables (e.g., pool size, coverage, number of bulks, cases of misclassification and different statistical algorithm). The results of our computer simulation experiment are discussed in the Supplementary Note 1 (Supplementary Fig. 5 ). Table 1 Identified genomic intervals for four agronomic traits Full size table Cloning and functional analysis of the QTL OsMADS1 GW3p6 In our previous study, we mapped a genomic region containing the QTL GW3p6 contributing to the high grain production of the elite hybrid rice variety Guang-Liang-You 676 (GLY-676) from F 2 individuals [16] . To further fine clone the QTL GW3p6 , we applied GPS to the F 2 population derived from the elite hybrid rice variety GLY-676 (heterozygous first filial (F 1 )), which was generated from a cross between the varieties FH (male line) and GZ (female line). First, we selected 1000-grain weight (TGW) as the trait for mapping heterotic genes. We ranked three categories (22.33–29.15 g/1000-grain, 29.16–31.09 g/1000-grain and 31.10–37.3 g/1000-grain) to phenotype TGW according to traits and then created simulated pools with their sequencing reads (individual sequencing reads data from European Nucleotide Archive under the accession number PRJEB13735). We implemented Ridit analysis with allelic frequencies from three bulks to calculate p values for each SNP (Fig. 2a ). As numerous background noises complicated locating the QTL at a fine resolution, a noise reducing strategy followed the statistical test. After conducting all analysis, we located a 400-kb candidate interval contributing to grain weight (Fig. 2b ). The mapping accuracy and resolution of GPS can reach almost the same level as that of Composite Interval Mapping. Notably, the GPS mapping results show that the method can be used as a faster and more convenient approach than conventional mapping methods in rice breeding. Considering the compatibility of the different versions of the assembled data, we remapped the TGW genes by GPS method based on Os-Nipponbare-Reference-IRGSP-1.0 (ref. [37] ) and MH63RS2 (ref. [38] ), and the genetic mapping results from the three reference genome assemblies were almost the same (Supplementary Fig. 6 ). Fig. 2 QTL mapping and map-based cloning of OsMADS1 GW3p6 . a , b Identification of the genomic region consisting of OsMADS1 GW3p6 via GPS approach. a The p value plot is the result of Ridit analysis for 1000-grain weight before noise-reduction algorithm. The -ln ( p value) plot ( Y axis) is plotted against SNP positions ( X axis) on each of the 12 rice chromosomes. b After the strategy of reducing background noise, the results present as ratio plot. X -axis value is set at a midpoint at each defined genomic interval and Y -axis value corresponds to ratio. c The genotype of chromosome 3 of RIL-79. Black, white and gray bars represent the heterozygous genotype, and homozygous genotypes of GZ and FH respectively. d In the fine-scale mapping (lower bar) generated from the analysis of 1,079 segregating individuals, the QTL GW3p6 falls in the heterozygous interval. The numbers below the bar indicate the number of recombinants between GW3p6 and the molecular markers shown. e Genotyping of progeny homozygous for GW3p6 delimited the locus to a ~5.9 Kb genomic region between markers MP99 and MP100. f , h 1000-grain weight and grain length of recombinant F 2 lines of RIL-79 (L1-L4). Data shown as means ± SD, n = 48. Source data are provided as a Source Data file. g Schematic diagram depicting the structure of OsMADS1 and OsMADS1 GW3p6 , red letters stand for the nucleotides of OsMADS1 non-homozygous segment. i The sequencing electrophoresis of non-homologous segment between OsMADS1 and OsMADS1 GW3p6 . j The schematic illustration of OsMADS1 functional domains, M represents the MADS domain, I represents the intervening domain, K represents the keratin-like domain, and C represents the C-terminal domain. Source data of Fig. 2f, h are provided in a Source Data file Full size image Furthermore, we screened the recombinant inbred lines (RILs) from the self-pollination F 5 generation, and RIL79, one RIL in which genomic segment of GW3p6 was heterozygous but others were homozygous, was selected as a further segregating population (Supplementary Fig. 7 ). We used 1,079 plants from the F 1 population of RIL79 to fine-scale map GW3p6 , and 36 SNP markers were used for genotyping, ultimately narrowed down the interval to a ~5.9-kb region flanked by MP99 and MP100 (Fig. 2c–h ). This region contains only the second half of Os03g0215400 (RAP-DB), and further sequencing analysis indicates a 15-bp non-homologous segment at the junction of the seventh intron and eighth exon of Os03g0215400 (Fig. 2g, i ), from TCCTTGGTGAAGGTA to ATGTATATATACT. The 3′ terminal bases AG of the seventh intron were altered, and we speculated that this might lead to alternative splicing. The cDNA sequencing data showed that the splice site (AG/GT) slipped to the 32nd nucleotide (AG/GC) of the last exon (Supplementary Fig. 8 ), directly caused a premature stop codon, and the original mature protein was truncated by 32 amino acid resides (Fig. 2j , Supplementary Fig. 9 ). We used the Insertion/Deletion (InDel) marker CS-92 to verify the association between grain size and alternative splicing. Totally 200 individuals of each OsMADS1 genotype were counted, and the heavier grain weight and more slender grain size were in complete agreement with OsMADS1 GW3p6 (Supplementary Fig. 10 ). These results are also consistent with the performance of three GW3p6 genotypes in the F 2 generation as previously reported [16] , and heterozygous OsMADS1 GW3p6 showed incomplete dominance. These results indicate that this OsMADS1 GW3p6 alternative splicing caused by non-homologous segment is responsible for significant grain weight as previously reported [39] , [40] . To further examine whether the function of OsMADS1 GW3p6 acted as a grain size gene, we transformed FH (male parent) with either rice Ubiquitin promoter-driven OsMADS1 cDNA from FH (p Ubi :: OsMADS1 -FH,OE- OsMADS1 ) or OsMADS1 GW3p6 cDNA from GZ (p Ubi :: OsMADS1 GW3p6 -GZ,OE- GW3p6 ). The grains of the p Ubi :: OsMADS1 GW3p6 transgenic plants were longer and heavier than the non-transgenic control plants (Fig. 3a–c ), but constitutive expression of the FH OsMADS1 cDNA driven by the rice Ubiquitin promoter led to abnormalities in lemmas and paleae, as previously described [41] , [42] (Fig. 3a ). Moreover, we designed the target primers at the last exon of OsMADS1 using the CRISPR-Cas9 system in FH (CR-FH). Sequencing analysis revealed several insertions and deletions at the last exon in transgenic plants that resulted in loss of function in the C domain of the protein encoded by OsMADS1 . The transgenic panicles exhibited phenotypic alterations (Fig. 3a ), including elongated leafy paleae and lemmas, as well as low fertility seriously as previously reported [40] , [42] . The result was also similar to the reported phenotype of leafy hull sterile 1 [41] . Furthermore, the C-terminal function caused changes in glume development. In addition, we transferred the same overexpression construct of OsMADS1 GW3p6 and knockout construct by CRISPR/Cas9 system to the japonica variety Nipponbare (NPB) with same OsMADS1 genotype as FH. The overexpressing NPB plants (OE- GW3p6 -NPB) exhibited longer and heavier grains compared with the non-transgenic plants (Supplementary Fig. 11c, d, e ). The transgenic NPB plants carrying missense mutations in the C domain of OsMADS1 (CR-NPB) exhibited the same phenotype as CR-FH plants (Supplementary Fig. 11a, b, c ). The above data imply that OsMADS1 plays a significant role in the development of rice flower. Typically, the C domain of OsMADS1 is closely related to the growth of glumes and the development of floral organs, and the function of OsMADS1 GW3p6 is to increase grain length and weight. Fig. 3 The phenotype of FH transgenic plants. a The grain morphology of FH and transgenic plants. FH represents the grain morphology of non-transgenic plant FH. CR-FH represents the grain morphology of transgenic FH plants containing missense mutations in C domain of OsMADS1 . OE- OsMADS1 represents the grain morphology of transgenic FH plants containing overexpression OsMADS1 construct. OE- GW3p6 represents the grain morphology of transgenic FH plants containing overexpression OsMADS1 GW3p6 construct. Scale bar, 5 mm. b Grain length in transgenic overexpression plants and non-transgenic plants. OE- GW3p6 -#1 and OE- GW3p6 -#2 indicate the two transgenic lines containing overexpression OsMADS1 GW3p6 construct. c 1000-grain weight in transgenic OsMADS1 GW3p6 overexpression plants and non-transgenic plants. Data in ( b , c ) are given as means ± SD ( n = 24) with the indicated significance by using a two-tailed Student’s t -test (** p < 0.01). Source data of Fig. 3b, c are provided as a Source Data file Full size image OsMADS1 encodes an MIKC c -type MADS-box transcription factor [43] ; it is also an E-class gene involved in rice floral organ development [44] , [45] . The MIKC-type MADS-domain proteins consist of four domains: the MADS domain, Intervening domain, Keratin-like domain and C Domain respectively. The C-terminal region has been associated with transcriptional activation [46] , and the non-homologous segment of OsMADS1 GW3p6 was located within the C domain. Therefore, we conducted transcriptional activation experiment by yeast one-hybrid system (Supplementary Fig. 12 ). The results showed that both full-length OsMADS1 and OsMADS1 GW3p6 had no transcriptional activity, which may be associated with a full-length inhibition of its transcriptional activity [46] . In addition, the transcriptional activity of the OsMADS1 C-terminal region was higher than that of OsMADS1 GW3p6 . To further verify our experimental results, we applied a fluorescence report system for transcription activation experiments in rice protoplasts. The results were consistent with the data obtained in the yeast system, with OsMADS1 showing approximately 5 times stronger transcriptional activity than OsMADS1 GW3p6 (Supplementary Fig. 13 ). These data were also consistent with previous reports that alternative splicing attenuates the activation of downstream genes, possibly regulating the transcriptional level of downstream auxin-related genes to change the grain size [39] . The analysis of rice young panicles through RT-qPCR indicated that the expression of OsMADS1 GW3p6 was indeed higher than OsMADS1 (Supplementary Fig. 14 ). According to our analysis of the structure of OsMADS1 GW3p6 , a large number of SNPs and InDels are located the upstream of the 5′UTR, and we evaluated whether the observed changes in expression are associated with nucleotides differences in the promoter. To this end, we used the fluorescence report system to verify the promoter, and found no obvious difference between the promoter of OsMADS1 and OsMADS1 GW3p6 (Supplementary Fig. 15 ). Thus, this change in expression was likely caused by a premature stop codon due to alternative splicing. Taken together, these changes in the C domain may have resulted in the change of grain size. Improved grain yield by constructing a NIL containing GW3p6 To further investigate the genetic function of GW3p6 , the near-isogenic line NIL-FH:: GW3p6 was generated by introgression of GW3p6 in the FH background. Some RILs with the genetic background of FH accounting for the vast majority were selected as backcrossing materials to generate NILs and were backcrossed twice to FH. With the aid of screening using a large number of molecular markers, and ultimately through sequence-based high-throughput genotyping, we generated a NIL with the FH genetic background and a ~130-kb heterozygous segment. Meanwhile, due to the heterozygous genotype on GW3p6 , we can observe phenotypic changes in the three GW3p6 genotypes among the offspring, and the phenotype of incomplete dominance could be observed (Fig. 4b ). In general, the phenotypes of NIL-FH:: GW3p6 were similar to that of FH (Fig. 4a ), including grain width, panicle number, panicle length, seed-setting rate, grain number per panicle and plant height (Fig. 4d, g–k ), though the grain length and 1000-grain weight of NIL-FH:: GW3p6 were ~6–7% higher than those of the FH plants (Fig. 4c, e ). In addition, the grain yield per plant of NIL-FH:: GW3p6 was increased by more than 8% (Fig. 4f ), while the heading date had a 1~2 days delay compared to that of FH (Fig. 4l ). Thus, GW3p6 is a useful target gene in breeding. By constructing a NIL, we demonstrated that an introgression line harboring a heterosis gene from the maternal parent could achieve better performance than inbred line. It also proved rice heterosis genes’ incomplete dominance played an important role in hybrid rice (Fig. 4b ). Fig. 4 A yield-related traits of FH and NIL-FH: GW3p6 . a Plant phenotype of FH and NIL-FH:: GW3p6 . Scale bar, 10 cm. b Grain morphology of FH, NIL-FH: GW3p6 and FH/ NIL-FH:: GW3p6 . NIL and FH represent the grain morphology of NIL-FH:: GW3p6 and FH, respectively. FH/NIL indicates the grain morphology of plants with heterozygous OsMADS1 ( OsMADS1/OsAMDS1 GW3p6 ) genotype. Scale bar, 5 mm. c – l A field-based comparison of the FH and NIL-FH:: GW3p6 plants. c Grain length, d grain width, e 1000-grain weight, f grain yield per plant, g panicle length, h panicle number, i seed-setting rate, j grain number per panicle, k plant height, and l heading date. Data are shown as means ± SD ( n = 24) with the indicated significance from a two-tailed Student’s t test. For statistical significance, * p < 0.05, ** p < 0.01, NS not significant. Source data of Fig. 4c–l are provided as a Source Data file Full size image The heterosis effect of OsMADS1 GW3p6 in rice breeding As shown above, the NIL carrying the heterotic gene OsMADS1 GW3p6 showed significantly increased grain yield. To further explore the potential of OsMADS1 GW3p6 in rice breeding, we pyramided another previously reported heterotic QTL PN3q23 underlying panicle number [16] . The plants harboring two heterotic genes exhibited ~15% increased grain yield compared to the FH plants (Fig. 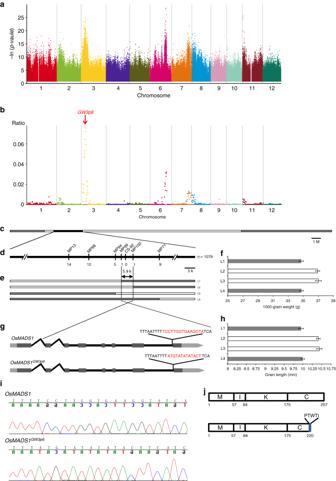Fig. 2 QTL mapping and map-based cloning ofOsMADS1GW3p6.a,bIdentification of the genomic region consisting ofOsMADS1GW3p6via GPS approach.aThepvalue plot is the result of Ridit analysis for 1000-grain weight before noise-reduction algorithm. The -ln (pvalue) plot (Yaxis) is plotted against SNP positions (Xaxis) on each of the 12 rice chromosomes.bAfter the strategy of reducing background noise, the results present as ratio plot.X-axis value is set at a midpoint at each defined genomic interval andY-axis value corresponds to ratio.cThe genotype of chromosome 3 of RIL-79. Black, white and gray bars represent the heterozygous genotype, and homozygous genotypes of GZ and FH respectively.dIn the fine-scale mapping (lower bar) generated from the analysis of 1,079 segregating individuals, the QTLGW3p6falls in the heterozygous interval. The numbers below the bar indicate the number of recombinants betweenGW3p6and the molecular markers shown.eGenotyping of progeny homozygous forGW3p6delimited the locus to a ~5.9 Kb genomic region between markers MP99 and MP100.f,h1000-grain weight and grain length of recombinant F2lines of RIL-79 (L1-L4). Data shown as means ± SD,n= 48. Source data are provided as a Source Data file.gSchematic diagram depicting the structure ofOsMADS1andOsMADS1GW3p6, red letters stand for the nucleotides ofOsMADS1non-homozygous segment.iThe sequencing electrophoresis of non-homologous segment betweenOsMADS1andOsMADS1GW3p6.jThe schematic illustration ofOsMADS1functional domains, M represents the MADS domain, I represents the intervening domain, K represents the keratin-like domain, and C represents the C-terminal domain. Source data of Fig.2f, hare provided in a Source Data file 5a , Table 2 ), as well as higher yield than NIL-FH:: GW3p6 plants (Table 2 ). The panicle number of the plants harboring PN3q23 was also significantly increased compared with that of FH (Supplementary Table 2 ). We measured the yield per plant for FH, NIL-FH:: GW3p6 and GLY676 respectively. The results exhibited that GW3p6 explained 27.8% of the heterotic effect (Fig. 5b ). The GW3p6 and PN3q23 , two major heterotic genes from the female parent, explained over 40% of the heterotic effect (Fig. 5b ). These findings implied a few heterotic genes from female parent played important roles in heterosis. We detected the haplotype of OsMADS1 GW3p6 in 1328 varieties of hybrid rice (Supplementary Data 1 ) simultaneously. OsMADS1 GW3p6 was rarely detected among the three-line type hybrids, in which the proportion was ~1.6%. Approximately 11.5% of the two-line type hybrid varieties were found to carry the OsMADS1 GW3p6 allele. These data indicate there is a large breeding potential for application of the superior allele of OsMADS1 GW3p6 in future hybrid rice breeding. Fig. 5 The heterosis effect of OsMADS1 GW3p6 in rice breeding. a The phenotype of FH plants and plants carrying two heterotic genes GW3p6 & PN3q23 . Scale bar, 10 cm. b The yield-related contribution of GW3p6 and PN3q23 . The proportion of GW3p6 and PN3q23 in yield-related heterosis effect are indicated in the pie chart. The color red and orange represent the heterosis contribution rate of GW3p6 and PN3q23 respectively. The color blue indicates the heterosis contribution rate of heterotic genes exclude GW3p6 and PN3q23 . c The flow chart of improvement breeding about hybrid rice in this study. d The strategy of rice-improvement breeding in conventional rice and hybrid rice. Colored circles represent superior alleles, for example, the blue, purple and brown circles denote superior alleles associated with tiller number, panicle type and plant architecture. Souce data of Fig. 5b are provided as a Source Data file Full size image Table 2 Grain yield per plant of different plants harboring heterosis genes Full size table In conclusion, the heterotic gene GW3p6 can improve the grain yield significantly in hybrid rice. By dissecting the heterotic gene OsMADS1 GW3p6 , we summarized a rice breeding strategy in hybrid rice and inbred rice (Fig. 5c, d ). The F 1 progeny derived from different crosses exhibited heterosis in certain agronomic traits, and we could locate superior genes in their F 2 generations through the rapid and convenient GPS method, finally achieving fast and precise breeding through the marker-assisted selection approach. Traditional QTL mapping methods depending on the genetic linkage of QTLs to visible makers are laborious and time-consuming. The advent of NGS technologies and BSA has offered new opportunities for rapid identification of QTLs. Several methods have been established to accelerate the works in genetic mapping. We developed GPS, an improved approach combining high-throughput sequencing with modified BSA, for QTL mapping in crop breeding. Our method has several advantages over several previous methods. First, instead of using mutant lines such as Mutmap [26] and Next-generation mapping [28] , we choose parental lines comprising a large quantity of useful alleles directly. Second, our approach only requires F 2 generation, reducing a great amount time needed for constructing genetic population. Third, GPS has a high resolution of ~400-kb, whereas the resolution of QTL-seq [29] is ~2 Mb. In this work, we successfully identified the QTLs underlying five target traits (heading date, plant height, tiller angle, flag leaf angle and grain weight) in rice, demonstrating that GPS has a robust and extensive applicability for QTL mapping. In addition, the cost-effectiveness of the entire GPS process is relatively high compared with other methods. With the decline in high-throughput sequencing, applying GPS to identify QTLs would be economical. GPS can map QTLs underlying multiple traits simultaneously in one rice population. For example, a leaf sampled once can be used multiple times. Moreover, GPS does not require genotyping of all individuals, saving both time and laborious effort. Overall, this method significantly enhances the efficiency and cost-effectiveness of mapping candidate genes, enabling rapid identification of heterotic genes for rice breeding. Breeders and researchers would find good trade-offs in cost-effectiveness due to the relatively broad requirements and high efficiency of GPS. Thus, the highly efficient GPS will dramatically accelerate crop improvement in a cost-effective manner. GPS shows a relatively wide range of applications in fine-mapping and breeding, but some limitations are also existed in GPS approach. First, QTL by environment interaction (QEI) is widely present in crops and other species. GPS with Ridit analysis currently had low power in QEI. Second, the GPS pipeline may not work very well with the overdominant loci. To identify QTLs through the software GPS, the SNPs related to the agronomic traits need to have a great distinction of reference reads to alternative reads. However, for the overdominant loci, there may be a great distinction of heterozygous genotypes to homozygous genotypes, but less great distinctions of reference reads to alternative reads. These limitations of GPS should be accounted for and assessed in plant breeding and fine mapping. In our simulation experiment, we consider five experimental variables that influence the results of accurate detection. In the first place, we took the possibility that unlinked SNPs were calculated as related one into consideration. The simulation indicated that the number of individuals in each bulk had an impact on it. The more individuals we selected in each group, the less likely errors of false positive occurred. Furthermore, the number of pools is another important variable in our method. Meanwhile, more bulks meant being less influenced by incorrect categorization, thus we needed a balance here. In the simulation of the effects of misclassification, we took the 20% wrong classification of individuals in a certain bulk as an example, and this would be the main element leading to the inaccuracy of results. Three factors, depth, number of selected individuals and number of bulks, together influenced the capability of our method to detect the QTL within the context of misclassification. With the increasing value of these experimental variables (depth, pool size, number of bulks), the power to uncover the QTLs becomes larger. Finally, we also assessed the results of different statistical algorithms and determined the optimal one. It turned out that the Ridit analysis had the best performance in identifying QTL among them. As shown above, the near isogenic line NIL-FH:: GW3p6 displayed a large increase in yield compared with FH, but it was still slightly less productive than the F 1 plants. The reason for this phenomenon is mainly there are multiple heterosis genes from maternal parents. With the benefits of accurate QTL mapping, GWAS and an improved GPS tool will be able to rapidly identify heterotic genes for crop breeding. Further studies are needed to identify and pyramiding more heterotic genes with regard to various yield-related traits in important backbone parent, such as the tiller number related gene PN3q23 . The incomplete dominance effect of OsGW3p6 may be due to an allelic dosage effect as in maize [47] . Uncovering more alleles and fine-tuning the dosage of OsMADS1 GW3p6 may produce an optimal yield as previously study in tomato [48] , [49] . To explore the potential of rice breeding, we also sequenced the genome DNAs of hybrid rice parents (Supplementary Data 2 ). The results showed that in two-line hybrid rice, there are three male-sterile lines carried OsMADS1 GW3p6 , i.e., M6303S, Xuan69S and Guangzhan63S. In three-line hybrid rice, the proportion of OsMADS1 GW3p6 is small. Moreover, OsMADS1 GW3p6 was present in the restorer line, such as Nanhui511, a big spike-type indica restorer line with broad adaptability. A phylogenetic tree of 1,473 indica-indica hybrid rice varieties showed that over half of those containing OsMADS1 GW3p6 were clustered with the hybrid rice GLY-676 (Supplementary Fig. 16 ), which may be associated with a similar genotype grouped in the same clade. Using rice pan-genome data [50] , we found that OsMADS1 GW3p6 mainly existed in the tropical japonica varieties among 66 rice accessions (Supplemental Fig. 17 ). These data indicate that OsMADS1 GW3p6 has not been exploited in large-scale rice breeding and that the OsMADS1 GW3p6 allele has great potential in rice breeding, particularly in hybrid rice. Either as a male-sterile line or restorer line, O sMADS1 GW3p6 will have a huge impact on rice breeding. In order to meet the growing demand, rice hybrid breeding requires additional superior germplasm resources to enhance yield potential, and future molecular breeding will need to overcome inter-subspecific hybrid sterility to broaden genetic diversity and enhance heterosis [51] , uncovering more heterotic genes for use in molecular breeding. We believe the GPS method and rice-improvement breeding strategy reported here will promote hybrid rice breeding. Plant materials and trait measurement In the GPS study, four sets of elite hybrid rice were used as mapping populations. The F 2 generations were obtained by self-pollinating F 1 hybrid rice. The F 2 populations with a large range of phenotypic variations were used for identifying QTLs for four agronomic traits (plant height, heading date, flag leaf angle, tiller angle). The four sets of F 2 populations were planted in a rice paddy located in Hainan Province during the standard growing season, and phenotypic investigations in the field were conducted in the appropriate growth stage in spring of 2017. In the fine-mapping study, Fuhui676 (FH), an elite indica restorer line, and the Photo-Thermo Sensitive Genic Male Sterile Line Guangzhan63-4S (GZ) were used as the recurrent and donor parent respectively, to develop the backcross population and NILs. The RILs that the genetic background of FH accounts for the vast majority were selected as backcross materials to generate NILs. In particular, RIL-81, an F 6 RIL derived from the cross between FH and GZ, carries a heterozygous segment harboring OsMADS1 GW3p6 . RIL-81 was backcrossed twice to FH. By screening a large number of molecular markers, and ultimately through sequence-based high-throughput genotyping, we generated the FH genetic background NIL-FH:: GW3p6 containing a ~130-kb heterozygous segment. Similarly, allelic combinations of OsMADS1 GW3p6 and PN3q23 were selected from the cross NIL-FH:: GW3p6 and Chromosomal Segment Substitution Line containing the PN3q23 segment. All of the plant materials were cultivated in the experimental field in Shanghai in summer or Sanya in winter. Field-grown NIL plants and gene pyramiding plants were grown in a rice paddy at an interplant spacing of 30 × 16 cm during the standard growing season at experimental fields located in Sanya (Hainan Province, China). Grain length and width were measured using an automatic digital grain size scanner, and fully filled grains were used for measuring 1000-grain weight. Ten plants in the middle of each row were harvested individually and used to investigate yield-related traits, such as panicle number and grain weight per plant. The phenotype data for plant height, panicle length, grain number per panicle and seed-setting rate were obtained using the main culm of each plant. The phenotype of NIL-FH:: GW3p6 plants was investigated in spring of 2018 in Hainan, China. The phenotype of plants containing GW3p6 and PN3q23 was investigated in autumn of 2018 in Shanghai, China. Bulked-segregant analysis To validate our method, we chose four complex traits to conduct proof-of-principle experiments. As illustrated in Supplementary Table 1 , four agronomic traits were observed in the four sets of F 2 populations. For plant height, according to phenotypic values, we classified F 2 populations into several bulks from high to low plant height. The same strategy was carried out with the other three traits using their F 2 progeny. The number of pools depends on the grade of the phenotypic difference and the number of F 2 individuals. The phenotypic values of F 2 individuals were arranged in ascending or descending order. The F 2 individuals corresponding to the phenotypic grade were marked and assigned to different pools. In the process of identifying heterotic gene GW3p6 , we divided the individuals into three ordinal pools according to 1000-grain weight (22.33–29.15 g/1000-grain, 29.16–31.09 g/1000-grain, 31.10–37.3 g/1000-grain), and pool size was 351 (33.56% of the total F 2 individuals), 348 (33.27%) and 347 (33.17%), respectively. Whole-genome sequencing of bulked DNA For each pool, genomic DNAs were extracted from the fresh leaf tissue of F 2 individuals using DNeasy Plant Mini Kit (Qiagen). The equal masses of fresh leaves (~0.05 g) were used for DNA pool sequencing. Equal masses of fresh leaves from F 2 individuals in each pool were mixed in a mortar, and then the genomic DNA of them was extracted for further sequencing. After that, the genomic DNA was fragmented by ultrasonic treatment. A sequencing library was constructed with an insert size of 400–500 bp for a single index according to the protocol of KAPA Hyper Prep Kit (Illumina ® platforms). The indexed DNA samples of each pool were then purified using a silica membrane column, followed by size-selection agarose gel electrophoresis (Bluepinpin). The DNA library of each pool was loaded into one lane using the Illumina Hiseq2500 system. In total, 2889 individuals in 37 lanes were sequenced, generating 100-bp paired-end reads. Alignment against the reference genome sequence (IRGSP releases build 4.0 pseudomolecules of rice; Os-Nipponbare-Reference-IRGSP-1.0; MH 63RS2) was performed using BWA software [33] , followed by SNP-calling using GATK [34] Best Practices ( https://software.broadinstitute.org/gatk/best-practices/ ). Filtering process for the sequencing data Before applying statistical tests to sequencing data, filtering process should be accomplished to guarantee accuracy. The four aspects of filtering criteria are as follow: (1) filtering out of low-quality variants; (2) selecting variants with appropriate depth; (3) screening out variants for which both parental lines present homogeneous and different genotypes; (4) filtering out of the SNPs for which sequence reads from all pools only showed non-reference bases. Statistical analysis was then applied to reveal causative variants. Applying statistical test After filtering process, we coped with sequencing data by statistical tests. Comparing with three nonparametric methods here, Ridit analysis [32] , Kruskal-Wallis Test [52] , and Chi-square test [53] , we chose the optimize one-Ridit analysis. Calculating p value of each variant, we pictured p value plot by using –ln ( p value) and chromosomal position as y -value and x -value, respectively. Reducing background noise scheme Even though we obtained the p value of each variant, this was not enough to pinpoint the QTL intervals. We implemented a reducing background noise scheme. Computing the ratio of number of statistically significant variants to total number of variants in a defined interval (~400-kb), while skipping interval where the number of total SNPs is less than 10. We identified the candidate genetic intervals responsible for phenotype via ratio plot. The location of peak represents a cluster of highly linked variants to a given trait in this 400-kb region. Genotyping and fine mapping of OsMADS1 GW3p6 Plant materials’ genotyping were mainly based on Applied Biosystems 3730 XL fully automatic DNA sequencer to identify SNPs, and high-throughput genotyping by whole-genome resequencing was used to confirm the background genotype [54] . The high resolution melting curve analysis by Roche LightCycler 480 and other genotyping methods (SNPs genotyping by Sanger Sequencing and InDels genotyping by gel electrophoresis) were used to genotype for constructing NIL-FH:: GW3p6 . Fine-scale mapping of OsMADS1 GW3p6 was based on 1,079 F 1 individuals of RIL-79. 36 SNP markers were used to screen the recombinants. Finally, the OsMADS1 GW3p6 locus was narrowed down to a 5.9-kb region between markers MP99 and MP100. The phenotype of grain shape and grain weight in selected recombinants was confirmed using the self-progeny test. The genomic DNA of candidate OsMADS1 genes from GZ, FH and other landrace varieties were sequenced and analyzed by Sanger Sequencing System. 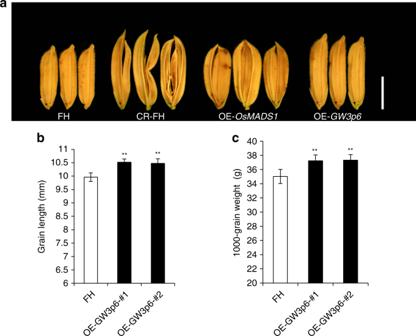Fig. 3 The phenotype of FH transgenic plants.aThe grain morphology of FH and transgenic plants. FH represents the grain morphology of non-transgenic plant FH. CR-FH represents the grain morphology of transgenic FH plants containing missense mutations in C domain ofOsMADS1. OE-OsMADS1represents the grain morphology of transgenic FH plants containing overexpressionOsMADS1construct. OE-GW3p6represents the grain morphology of transgenic FH plants containing overexpressionOsMADS1GW3p6construct. Scale bar, 5 mm.bGrain length in transgenic overexpression plants and non-transgenic plants. OE-GW3p6-#1 and OE-GW3p6-#2 indicate the two transgenic lines containing overexpressionOsMADS1GW3p6construct.c1000-grain weight in transgenicOsMADS1GW3p6overexpression plants and non-transgenic plants. Data in (b,c) are given as means ± SD (n= 24) with the indicated significance by using a two-tailed Student’st-test (**p< 0.01). Source data of Fig.3b, care provided as a Source Data file 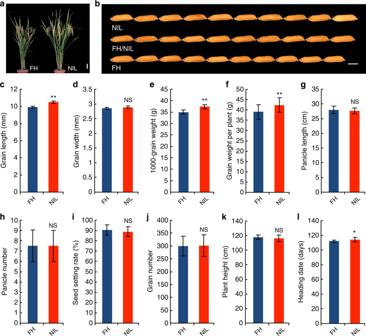Fig. 4 A yield-related traits of FH and NIL-FH:GW3p6.aPlant phenotype of FH and NIL-FH::GW3p6. Scale bar, 10 cm.bGrain morphology of FH, NIL-FH:GW3p6and FH/ NIL-FH::GW3p6. NIL and FH represent the grain morphology of NIL-FH::GW3p6and FH, respectively. FH/NIL indicates the grain morphology of plants with heterozygousOsMADS1(OsMADS1/OsAMDS1GW3p6) genotype. Scale bar, 5 mm.c–lA field-based comparison of the FH and NIL-FH::GW3p6plants.cGrain length,dgrain width,e1000-grain weight,fgrain yield per plant,gpanicle length,hpanicle number,iseed-setting rate,jgrain number per panicle,kplant height, andlheading date. Data are shown as means ± SD (n= 24) with the indicated significance from a two-tailed Student’sttest. For statistical significance, *p< 0.05, **p< 0.01, NS not significant. Source data of Fig.4c–lare provided as a Source Data file A list of the markers used for fine-scale mapping and NIL construction were given in Supplementary Table 3 and Supplementary Table 4 . Plasmid construction and plant transformation To generate the overexpression vector, full-length coding sequence without the stop codon of OsMADS1 and OsMADS1 GW3p6 were cloned into the vector pNCGR-OX fused with His-tag. And to construct sgCRISPR-Cas9 vector, one CRISPR/Cas-mediated target in C-Domain was cloned into CRISPR/Cas9 vector [55] . All the constructs were transformed to japonica cv. Nipponbare and indica cv. FH by Agrobacterium-mediated transformation. 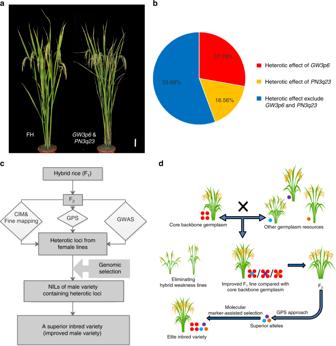Fig. 5 The heterosis effect ofOsMADS1GW3p6in rice breeding.aThe phenotype of FH plants and plants carrying two heterotic genesGW3p6&PN3q23. Scale bar, 10 cm.bThe yield-related contribution ofGW3p6andPN3q23. The proportion ofGW3p6andPN3q23in yield-related heterosis effect are indicated in the pie chart. The color red and orange represent the heterosis contribution rate ofGW3p6andPN3q23respectively. The color blue indicates the heterosis contribution rate of heterotic genes excludeGW3p6andPN3q23.cThe flow chart of improvement breeding about hybrid rice in this study.dThe strategy of rice-improvement breeding in conventional rice and hybrid rice. Colored circles represent superior alleles, for example, the blue, purple and brown circles denote superior alleles associated with tiller number, panicle type and plant architecture. Souce data of Fig.5bare provided as a Source Data file The relevant PCR primer sequences are given in Supplementary Table 5 . RNA extraction and quantitative RT-PCR analysis The total RNA was extracted from rice young panicles using TRIzol regent (Invitrogen), and 0.5 micrograms of total RNA was used to synthesize first-strand cDNA by the ReverTra Ace ® qPCR RT Master Mix with gRNA Remover (Code NO.FSQ-301, TOYOBO). Quantitative real-time PCR was performed from cDNA using THUNDERBIRD ® SYBR ® qPCR Mix (QPS-201, TOYOBO) according to the manufacturer’s instructions on Applied Biosystems Q5. The rice ubiquitin 5 gene was used as an internal control, and each qRT-PCR assay was performed at least three times in biological and technological replicates. The relevant PCR primer sequences are given in Supplementary Table 5 . Transcriptional activation assay in yeast The full-length and different truncations or deletions coding sequence of OsMADS1 and OsMADS1 GW3p6 were introduced into the pGBKT7 (Clontech) vector to fuse the GAL4 DNA-binding domain. The empty pGBKT7 vector was as negative control. Then the vectors were transformed into yeast strain AH109 and the clones were diluted to an absorbance of 1.0 (1/10, 1/100, 1/1000) at OD 600 . 15 μl of liquid culture was plated on the control medium and SD/-Leu-His-Ade-+ X-α-Gal medium for 3d at 30 °C. The transcription activation assays were conducted according to the Matchmaker GAL4 Two-Hybrid System 3 (Clontech) user manual. The relevant PCR primer sequences are given in Supplementary Table 5 . Dual luciferase transcriptional activation assay The C-Domain of OsMADS1 and OsMADS1 GW3p6 were introduced into pGE vector to construct the effector plasmid. The pGE vector was made from pGBKT7 and pRI101-AN (Takara), the GAL4-BD domain from pGBKT7 was inserted into the pRI101-AN driven by 35S promoter. The pGreen-DBmini vector containing upstream activation sequence was design as the reporter plasmid, and then effector plasmids and reporter plasmids were transformed into rice protoplasts. The empty pGE vector was used as a negative control. Each expression assay was performed at least three times in biological and technological replicates [56] . Transient expression assays of promoter activity The prompter fragments of OsMADS1 (~3.6 kb upstream sequence of the OsMADS1 ) and OsMADS1 GW3p6 (~3.9 kb promoter fragment of the OsMADS1 GW3p6 ) were amplified from FH and GZ respectively, and were inserted into pGreen II 0800-LUC vector containing the firefly luciferase gene and the Renilla gene [57] . The rice protoplasts were isolated from rice culm of 7~12 days after seeding. Each of the OsMADS1 promoter-LUC vector was used for transient transformation into rice protoplasts. And the empty pGreen II 0800-LUC vector transferred into rice protoplasts was as negative control. For rice protoplasts transformation, at least four independent transformations were performed for each sample [58] . The relative activity of LUC to REN luciferase was measured by luminometer. Calculation of heterotic contribution rate In total, 15 plants of GLY-676, and 70 plants of FH, NIL-FH:: GW3p6 and NIL-FH:: GW3p6 & PN3q23 were used to calculate the heterosis effect contribution rate. Heterosis contribution rate was obtained as follows: 
    Heterosis contribution rate = Y_NIL - Y_FH/Y_GLY676 - Y_FH
 (1) Y GLY676 represents the average yield per plant of GLY-676 (F 1 ), Y FH represents the average yield per plant of FH, Y NIL represents the average yield per plant of NIL-FH:: GW3p6 . Phylogenetic analysis The 1439 indica-indica phylogenetic trees were constructed by the published data [15] . The haplotypes of OsMADS1 were classified into two categories: OsMADS1 and OsMADS1 GW3p6 , the iTOL (version 4.2.4) [59] was used to display and annotate the phylogenic tree, the red annotation indicated the haplotype of OsMADS1 GW3p6 . Similarly, the neighbor-joining tree of the 66 rice accessions constructed by PHYLIP and the package MEGA5 was as known data. According to the haplotype of OsMADS1 , the haplotype of OsMADS1 GW3p6 was marked as an asterisk by iTOL in NJ-tree of 66 rice accessions. Reporting summary Further information on research design is available in the Nature Research Reporting Summary linked to this article.